Maximizing omnidirectional light harvesting in metal oxide hyperbranched array architectures The scrupulous design of nanoarchitectures and smart hybridization of specific active materials are closely related to the overall photovoltaic performance of an anode electrode. Here we present a solution-based strategy for the fabrication of well-aligned metal oxide-based nanowire-nanosheet-nanorod hyperbranched arrays on transparent conducting oxide substrates. For these hyperbranched arrays, we observe a twofold increment in dye adsorption and enhanced light trapping and scattering capability compared with the pristine titanium dioxide nanowires, and thus a power conversion efficiency of 9.09% is achieved. Our growth approach presents a strategy to broaden the photoresponse and maximize the light-harvesting efficiency of arrays architectures, and may lead to applications for energy conversion and storage, catalysis, water splitting and gas sensing. Solar cells are regarded as one of the most promising energy technologies that have the potential to meet our growing energy demands [1] . Among the various types of solar cells, dye-sensitized solar cells (DSSCs) emerged as a promising alternative to the conventional silicon solar cells owing to their high efficiency (~13%), low cost as well as ease of fabrication procedure [2] , [3] , [4] , [5] . At the heart of these solar cells is the anode material, which plays a pivotal role in the device performance. More recently, the synthesis of well-organized nanostructures such as the organized mesoporous TiO 2 films prepared using graft copolymer nanostructural polymers [6] , [7] , [8] , [9] , [10] , and some well-aligned one-dimensional (1D) nanostructures, such as nanowires (NWs), nanotubes, nanorods (NRs) and nanofibres, have stimulated intense research interest and attention owing to their potential advantages of rapid charge transport and efficient charge collection by means of providing short electrical pathways for rapid transfer and thus efficient collection of photo-generated carriers throughout the device [11] , [12] , [13] , [14] , [15] , [16] , [17] . It is well known that the key to high solar-to-electric efficiency is surface area. Nevertheless, for the 1D nanostructure-based electrode, a fundamental drawback is the insufficient internal surface area and thus low dye-loading capacity owing to a low roughness factor or the considerable free space between adjacent 1D nanostructures [18] , [19] . One of the approaches to increase the surface area for improving the device performance is to increase the length of 1D nanostructures [20] . Another classical solution is to decorate the 1D nanostructures with dendritic NR branches [21] , [22] , [23] . For example, several studies regarding long NWs or the assembly of 1D nanostructures into three-dimensional (3D) hierarchical tree-like or bush-like branched NW structures have been reported [24] , [25] , [26] , [27] , [28] , [29] . In this regard, the enhancement of surface area is still restricted along either the axial or ambient directions. However, a strategy that can maximize the surface area of 1D nanostructures across three dimensions by means of providing ample germination sites to anchor additional building units is still missing. 1D nanostructures have been viewed as an ideal scaffold to composite with other homogeneous or heterogeneous structures such as nanoparticles (NPs), NRs, nanosheets (NSs), nanotubes and so on in order to ensure high surface area, reinforce light scattering and trapping and suppress unexpected back reaction (charge recombination) [30] , [31] , [32] , [33] . In particular, 2D NSs have been regarded as promising nano-components that exhibit bifunctional properties of both large surface area for dye adsorption and relatively direct pathways for the transportation of electrons to the electrode [34] , [35] , [36] . TiO 2 is most commonly used as a photoanode in DSSCs, and to date, the best of state-of-the-art DSSC is based on the anatase TiO 2 anode materials. To the best of our knowledge, few successful examples regarding homogeneous hierarchical structures consisting of epitaxial TiO 2 NSs (TNSs) on vertically aligned TiO 2 NWs (TNWs) have been reported for solar cells, not to mention subsequent multi-linked NR branch germination. In this communication, a solution-processed method to construct oriented hierarchical isomeric TiO 2 hyperbranched array materials composed of three basic constitutional units, that is, NWs, NSs and NRs, on TCO substrates for high efficiency DSSCs is reported. Our design starts from vertically aligned anatase TNWs with smooth surfaces and loose alignment. The TNSs are epitaxially grown onto the TNW via a unique and effective acid-thermal reaction, which provides ample ‘active sites’ for additional NR branch germination onto the interstices of the well-aligned TNS and the free spaces of the TNW scaffolds. Via variation from pure 1D backbones to complex 3D monoblocks, the hyperbranched array (TNW–NS–NR) film exhibits substantially enlarged surface area, for which a twofold increase of the dye-loading capacity is observed compared with the parental TNW counterpart. Consequently, an enhanced absolute full-sun efficiency of 9.09% is attained for a TNW–NS–NR-based cell, which is 77% higher than the pure TNW-based device (5.15%) and 24% higher than the highest value reported for hierarchical TNWs based cell (7.34%) with a similar film thickness [23] . The enhancement could primarily arise from the synergistic effects of enlarged dye loading and improved light scattering, which maximize the light-harvesting capability of the array architectures. Preparation of various aligned array architectures The schematic illustrations and corresponding scanning electron microscopy (SEM) images of TiO 2 nanoarrays with three fundamentally different morphologies synthesized via successive hydrothermal/acid-thermal processing (seen in Supplementary Fig. 1 ) are shown in Fig. 1 . 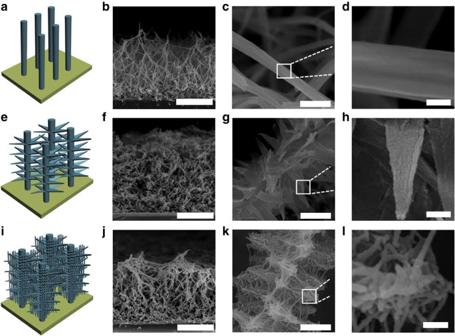Figure 1: Structure of TiO2nanoarrays. Schematic illustrations and SEM images of various TiO2nanoarrays on FTO glass substrate at low and high magnifications. (a–d) pristine TNW arrays with smooth surface. (e–h) TNW–NS branched arrays. (i–l) TNW–NS–NR hyperbranched arrays. Scale bar, 10 μm (b,f,j), 500 nm (c,g,k) and 100 nm (d,h,l). Figure 1: Structure of TiO 2 nanoarrays. Schematic illustrations and SEM images of various TiO 2 nanoarrays on FTO glass substrate at low and high magnifications. ( a – d ) pristine TNW arrays with smooth surface. ( e – h ) TNW–NS branched arrays. ( i – l ) TNW–NS–NR hyperbranched arrays. Scale bar, 10 μm ( b , f , j ), 500 nm ( c , g , k ) and 100 nm ( d , h , l ). Full size image Figure 1b,c shows SEM images of a cross-sectional view and corresponding individual NW, respectively. Obviously, a uniform and well-separated NW array with a smooth surface and a length of ~16 μm grow almost vertically from the substrate during a hydrothermal reaction for 3 h, confirming their preferential growth along the y -axial (001) direction over the x -axial (110) direction in the case of the potassium titanium oxide oxalate dehydrate (PTO)/H 2 O/diethylene glycol (DEG) hydrothermal system [23] . The prepared NWs show a bundle-like morphology consisting of several slim wires (~70–80 nm in diameter) ( Fig. 1d ), and the diameters are in the range of ~200–300 nm ( Fig. 1c ). Subsequently, the pristine NWs are processed to yield hierarchical NW–NS structures via a titanium isopropoxide (TTIP)/acetic acid (HAc) acid-thermal growth at 150 °C for 9 h (seen in the Methods section). Strikingly, the originally smooth NWs are distinctly converted into the hierarchical feature ( Fig. 1g ) with a large number of lamellar NSs uniformly and epitaxially constructed on the NWs surface in different angles to each other. It can be seen in Fig. 1h that such NSs show a textured and rough surface composed of well-connected nanocrystallites, which can provide a large surface area for dye adsorption. Also, considerable nanopores can be formed on the NSs, which are expected to be beneficial for the electrolyte diffusion. More importantly, the planar sheet-like shape can offer sufficient active sites for anchoring enormous number of branches. Afterwards, the as-fabricated NW–NS arrays undergo the third-step hydrothermal reaction again in the PTO/H 2 O/DEG system with another optimized hydrothermal condition profile, leading to highly branched nanostructures with a host of cross-linked NR branches (several nanometres in diameter and hundreds of nanometres in length) filling the interstice and voids between the adjacent NSs and the surplus space existing among the NWs scaffold ( Fig. 1k,l ). One can notice that the NRs tie the adjacent NSs together as well as the NWs trunk ( Fig. 1l ), and eventually all interweave into the well-interconnected porous pine-tree-like NW–NS–NR hyperbranched arrays. Such extremely complex 3D nanostructured arrays are believed to increase not only the surface area but also the light trapping and scattering ability, resulting in an enhancement of the light-harvesting efficiency of DSSCs. It is also apparent that the successive solution processing does not lead to a change of total film thickness ( Fig. 1f,j ); instead, a continuous evolvement from a 1D structure into a complex 3D hierarchical architecture can be witnessed. The prepared nanoarray photoanodes are all indexed as anatase phase TiO 2 (JCPDS No. 21-1272) as confirmed by X-ray diffraction (XRD) patterns in Supplementary Fig. 2 . It is worth noting that the intensity of (101) characteristic peak increases with the successive branch modification, indicating an improved crystallinity of hierarchical structures. Such a highly crystalline structure would effectively enhance the photovoltaic performance. The intrinsic morphological and structural properties of the as-prepared TiO 2 arrays are further characterized by transmission electron microscope (TEM) analysis. Supplementary Fig. 3 shows the basic TEM images of three different types of TiO 2 array architectures at a low magnification. As shown in Fig. 2a,b , the original TNWs are of relatively smooth surface without secondary structure. The NWs consist of several solidly packed NWs with diameter of ~70–80 nm. The high-resolution TEM image ( Fig. 2c ) together with the corresponding selected-area electron diffraction pattern (inset in Fig. 2c ) identify that NWs are single crystallites with a good crystallinity and a lattice spacing of 0.36 nm, which can be ascribed to the (101) planes of anatase TiO 2 . Close examination of these TNW–NS hierarchical structures reveals that a large number of NSs with a thickness of ~16 nm and length of 160–500 nm grow uniformly and epitaxially on the TNW surface ( Fig. 2d ). The magnified image indicates that individual NS is composed of numerous connected nanocrystallites with sizes of about 8–10 nm ( Fig. 2e ). 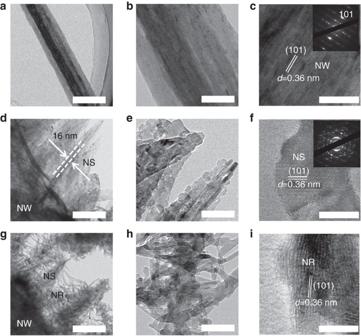Figure 2:TEM images of TiO2nanoarrays. (a–c) smooth TNW arrays. (d–f) hierarchical TNW–NS arrays. (g–i) TNW–NS–NR hyperbranched arrays. Inset images are the selected-area electron diffraction patterns. Scale bar, 200 nm (a,d,g), 50 nm (b,e,h) and 5 nm (c,f,i). Figure 2f and the inset selected-area electron diffraction images demonstrate the polycrystalline assembling nature of the anatase NSs. On the other hand, Fig. 2g–i illustrate omnidirectional coverage of high aspect ratio slender anatase NR branches (3–5 nm in diameter and 150–250 nm in length) on the NW and NS surfaces. These NR branches can not only effectively enlarge the surface area for higher dye loading, but also act as the bridge to link the adjacent NS and NW scaffolds, which can weave a 3D network to enhance light trapping and scattering of the array photoanodes. Figure 2: TEM images of TiO 2 nanoarrays. ( a – c ) smooth TNW arrays. ( d – f ) hierarchical TNW–NS arrays. ( g – i ) TNW–NS–NR hyperbranched arrays. Inset images are the selected-area electron diffraction patterns. Scale bar, 200 nm ( a , d , g ), 50 nm ( b , e , h ) and 5 nm ( c , f , i ). Full size image Growth mechanisms of arrays Time-dependent hydrothermal experiments are conducted to tailor systematically the TiO 2 structures and to scrutinize the growth process of the TNW–NS hierarchical array and TNW–NS–NR hyperbranched array structures. The resulting samples are examined by SEM analysis, and a schematic sketch showing the visual growth process is also displayed in Fig. 3m . For the assembly of TNW–NS hierarchical structures in TTIP/HAc acid-thermal reaction as clearly evidenced in Fig. 3a–f , a dense layer of TiO 2 NPs deposited uniformly in the initial stage (1 h, Fig. 3b ) on the original TNW surface, exhibiting a smooth-to-rough change, which results primarily from the initial hydrolysis of the TTIP precursor into NPs. Only after a certain period of time (3 h, Fig. 3c ) does the growth of lamellar and textured sheet-like structures on TNW scaffold take place. During this growth phase, ripe nanocrystallites connect and crystallize to form NS petals through an oriented attachment process in the presence of HAc [37] . As the hydrothermal reaction progressed to 6 h and over, both the number and length of NSs on the surface of TNW scaffold augment proportionately along with acid-thermal reaction time, for which numerous epitaxial NSs appear surrounding the TNW ( Fig. 3d,e ). As the growth time is further increased to 12 h, the TNW is entirely wrapped by a higher density of NSs ( Fig. 3f ). However, it is worth noting that the thickness of NSs is time invariant with a constant value of about 16 nm, while the length increase of NSs is not unlimited and the growth will terminate with the gradual decrease of Ti precursor concentration. The importance of the present work is that the difficulty of constructing thin anatase TNSs with epitaxial orientation on vertically aligned anatase TNW arrays has been overcome for the first time by such a simple and effective manner without pre-formation of a seed layer. While for the fabrication of TNW–NS–NR hyperbranched array architectures via subsequent hydrothermal treatment of TNW–NS in PTO/H 2 O/DEG mixed solution, the amount and length of the NR branches increase simultaneously along with the extension of hydrothermal reaction time ( Fig. 3g–l ), eventually leading to an interesting pine-tree-like morphology with luxuriant foliages. 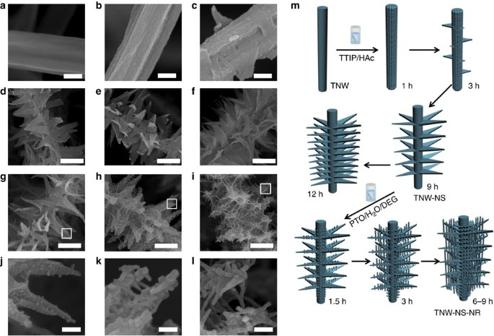Figure 3: Experimental and schematic representations of array growth. The time-dependent field emission SEM images and corresponding schematic sketches of growing hierarchical TiO2nanoarrays at different acid-thermal/hydrothermal conditions. (a–f) TiO2nanostructures after acid-thermal treatment of pristine TNW in TTIP/HAc system at 150 °C for 0, 1, 3, 6, 9 and 12 h, respectively. (g–l) TNW–NS–NR hyperbranched arrays prepared with TNW–NS under PTO/H2O/DEG hydrothermal system at 180 °C for 1.5, 3 and 9 h, respectively. (m) Schematic diagram showing the growth process of hierarchical TNW–NS and subsequent TNW–NS–NR hyperbranched arrays architectures. Scale bar, 100 nm (a–c,j–l) and 500 nm (d–i). Figure 3j–l shows clearly the variations of NR branches. Interestingly, the NRs dispersedly grown on the flat surfaces and side faces of the NSs in conjunction with their bridging effect on connecting the adjacent NSs could greatly increase the surface area and promote light scattering. Lastly, the successful construction of well-defined 3D complex TNW–NS–NR hyperbranched array structures and the robust contacts and connections among the TNW, TNS and TNR constituents should be attributed to the induced growth effects, matching lattices and interface of homogenous anatase TiO 2 . Figure 3: Experimental and schematic representations of array growth. The time-dependent field emission SEM images and corresponding schematic sketches of growing hierarchical TiO 2 nanoarrays at different acid-thermal/hydrothermal conditions. ( a – f ) TiO 2 nanostructures after acid-thermal treatment of pristine TNW in TTIP/HAc system at 150 °C for 0, 1, 3, 6, 9 and 12 h, respectively. ( g – l ) TNW–NS–NR hyperbranched arrays prepared with TNW–NS under PTO/H 2 O/DEG hydrothermal system at 180 °C for 1.5, 3 and 9 h, respectively. ( m ) Schematic diagram showing the growth process of hierarchical TNW–NS and subsequent TNW–NS–NR hyperbranched arrays architectures. Scale bar, 100 nm ( a – c , j – l ) and 500 nm ( d – i ). Full size image Photovoltaic performance and optical properties As-prepared vertically aligned TiO 2 array matrixes were then exploited as photoanodes to assemble DSSCs while the cells were irradiated by AM 1.5G simulated sunlight with a power intensity of 100 mW cm −2 . The preliminary photovoltaic performance test screening on the hierarchical photoanodes (TNW–NS) obtained by TTIP/HAc acid-thermal process for different reaction times (1, 3, 6, 9 and 12 h) or the hyperbranched TNW–NS–NR array photoelectrodes prepared in subsequent PTO/H 2 O/DEG hydrothermal process for different growth time (1.5, 3, 6 and 9 h) can be seen in Supplementary Tables 1 and 2 . 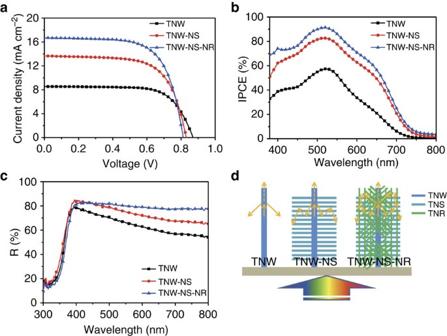Figure 4: Photovoltaic performance and optical properties. (a)J-Vcharacteristic and (b) Incident monochromatic photon-to-current conversion efficiency spectra of DSSCs based on TNW, TNW–NS and TNW–NS–NR array photoanodes with similar film thickness of 16 μm. (c) Diffused reflectance spectra and (d) schematic illustrations of light reflecting and scattering within the simplified network of TNW, TNW–NS and TNW–NS–NR array architectures. Figure 4a shows typical current density versus voltage ( J-V ) curves of three representative optimized TiO 2 samples, namely, TNW, TNW–NS (TTIP/HAc-9 h) and TNW–NS–NR (PTO/DEG/H 2 O-6 h), and the resultant photovoltaic parameters are summarized in Table 1 . It is apparent that the hierarchical configuration cells yield markedly enhanced efficiency (7.54% for TNW–NS and 9.09% for TNW–NS–NR) than their pristine TNW scaffold counterpart (5.15%), which predominantly results from significant enhancement of J sc . This result provides proof for the design concept of incorporating lamellar NSs and elongated NR branches onto all sides of TNW backbones so as to enhance the surface area for high dye loading. The as-prepared TiO 2 arrays showcase different geometry and porosity, and thus a different accessibility for dye adsorption. In order to qualify the area available for dye anchoring, the roughness factor measured by a N719 dye desorption method (as seen in Supplementary Table 3 ) [38] , [39] shows an increase of value from 516.0 to 1457.3 along with the continuously proceeded branched modification and thus indicating that the TNW–NS–NR hyperbranched arrays possess the largest surface area per unit volume for a given thickness for maximized dye uptakes. Hence, as seen in Table 1 , dye loading amount of approximately twofold increase for TNW–NS (97.77 nmol cm −2 ) and threefold increase for TNW–NS–NR (151.3 nmol cm −2 ) can be observed as compared with the TNW scaffold (53.57 nmol cm −2 ). Figure 4b displays the wavelength distribution of incident monochromatic photon-to-current conversion efficiency (IPCE) spectra of the DSSCs based on these three photoanodes. DSSC–TNW–NS and DSSC–TNW–NS–NR have higher IPCE values than that of DSSC–TNW over the whole spectral range from 400 to 800 nm, mainly due to the larger dye loading amount and more efficient light harvesting, resulting in a higher J sc , which is in concurrence with above J-V results. A broader photoaction in the red wavelength region observed in TNW–NS and TNW–NS–NR suggests that longer wavelength photons can be more efficiently converted to electrons, thus generating higher J sc . The light scattering and trapping as well as diffused reflectance properties of TiO 2 samples are evaluated with total and diffused transmittance and corresponding haze factor of the samples ( Supplementary Fig. 4 ), and the diffused reflectance spectra (seen in Fig. 4c ). Specifically, both the total and diffuse transmittances ( Supplementary Fig. 4a,b ) are reduced in the order of TNW>TNW–NS>TNW–NS–NR, while an increased portion of diffuse component in TNW–NS and TNW–NS–NR has been witnessed after the step-by-step branched modification, which could increase the overall characteristic size of the samples that can serve as the effective scattering elements [29] , [40] . Further evidence can be shown in the haze factor, which is plotted as a function of wavelength from 400 to 800 nm ( Supplementary Fig. 4c ). An increase order of TNW<TNW–NS<TNW–NS–NR in terms of haze factor is observed, indicating the increased portion of the transmitted light over the whole visible range can be scattered within complicated array architectures. Such hyperbranched array structures enable maximizing scattering efficiency, which would effectively multiply the optical path and increase the optical density within the TNW–NS and TNW–NS–NR photoanodes. On the other hand, compared with TNW, the TNW–NS and TNW–NS–NR with the hierarchical features exhibit higher reflectance capability and better scattering properties in the visible and near-infrared regions ( Fig. 4c ). Herein we propose the possible reflecting and scattering of light in a simplified matrix of TNW, TNW–NS and TNW–NS–NR ( Fig. 4d ). Apparently, the most complicated TNW–NS–NR architectures with multi-scale nature and interconnected network enable prominent optical confinement via multiple light reflections within the arrays and also are able to scatter the incident light of different wavelengths in the range of visible light [41] , [42] . This is conducive to extend the distance for light to travel within the photoelectrode, to induce more effective photon capturing in the visible region and thus resulting in an enhancement of light utilization efficiency [43] . Figure 4: Photovoltaic performance and optical properties. ( a ) J-V characteristic and ( b ) Incident monochromatic photon-to-current conversion efficiency spectra of DSSCs based on TNW, TNW–NS and TNW–NS–NR array photoanodes with similar film thickness of 16 μm. ( c ) Diffused reflectance spectra and ( d ) schematic illustrations of light reflecting and scattering within the simplified network of TNW, TNW–NS and TNW–NS–NR array architectures. Full size image Table 1 Photovoltaic parameters. Full size table The engineered integration of well-defined TNW, NS and NR components into a highly complex 3D monoblock (TNW–NS–NR hyperbranched arrays) resulted in a tremendous enhancement of J sc , which can be justified in three key ways: (1) a significantly enlarged surface area for higher dye loading resulting from sequential NSs and NRs modification; (2) a reinforced light trapping and scattering effect of the well-developed tree-like structure with luxuriant foliages and branches in a broad wavelength region; (3) the elongated and cross-linked NR branches serve as a bridge to connect the NSs anchoring sites and TNW scaffold, interweaving a porous fabric network, which can allow more efficient electrolyte diffusion and penetration into the interstice of the arrays. In other words, more effective photon capturing in the visible region and more dye molecules anchoring on the films will increase the probability of photon–dye molecule interaction, thus leading to high light-harvesting efficiency and high photo-generated current. Hence, an impressive efficiency of 9.09% was obtained for the devices based on TNW–NS–NR photoanodes of 16 μm in thickness, which is above the threshold for reported efficiency of devices fabricated similarly with N719 dye-sensitized TNW photoelectrodes of similar film thickness [23] . The details about the reproducibility of DSSCs with best performance are listed in Supplementary Table 4 , which further manifest the reproducibility of the current samples and performances are quite good and the results are reliable. Furthermore, in order to highlight the advantages of such TNW–NS–NR hyperbranched array-based cells, a fair comparison with the photovoltaic performance of the commercially available P25 TiO 2 NP (TNP)-based photoanode with a similar film thickness of ~16 μm was made. The detailed photovoltaic parameters are also denoted in Table 1 . The results indicate that both the J sc and V oc of TNW–NS–NR hyperbranched array-based DSSC are higher than that of the TNP counterpart, leading to an improved efficiency for the former. The enhanced J sc can be attributed to the superior light trapping and scattering efficiency for maximized light-harvesting efficiency and much more direct electron transit pathway for efficient electron transport within the TNW–NS–NR films with array architecture and geometry. The boosted V oc can be ascribed to its suppressed charge recombination and thus longer electron lifetime owing to its unique 1D wire trunk–2D sheet foliage–1D rod leave combined nanostructure with less grain boundaries and defects. Eventually, all of these advantageous factors lead to an impressive power conversion efficiency of TNW–NS–NR hyperbranched array-based DSSCs. Charge transfer and recombination dynamics Possible dissimilarity in the charge transfer and recombination dynamics within DSSCs arising from various TiO 2 structures are further characterized by intensity-modulated photocurrent/photovoltage spectroscopy (IMPS/IMVS). 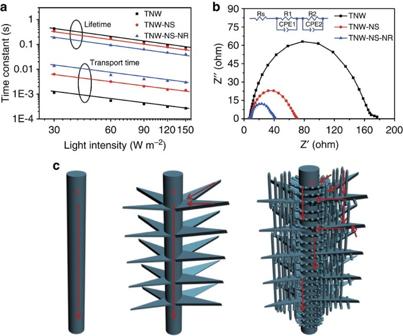Figure 5: Electron transfer and charge recombination dynamics. (a) Electron transport time and electron lifetime. (b) Nyquist mode plots of electrochemical impedance spectra of DSSCs based on TNW, TNW–NS and TNW–NS–NR array photoanodes with similar film thickness of 16 μm (inset is the simulated equivalent circuit). (c) Schematic demonstrations of electron transfer pathways for individual TNW, TNW–NS and TNW–NS–NR, respectively. Figure 5a shows the electron transport time ( τ d ) and lifetime ( τ r ) of three DSSCs obtained from IMPS and IMVS measurements, respectively, plotted as a function of light intensities [44] . Relative to smooth TNW-based cells, longer transport time (increased τ d ) and faster recombination rate (decreased τ r ) are obtained for hierarchical array-based devices (TNW–NS and TNW–NS–NR). Figure 5: Electron transfer and charge recombination dynamics. ( a ) Electron transport time and electron lifetime. ( b ) Nyquist mode plots of electrochemical impedance spectra of DSSCs based on TNW, TNW–NS and TNW–NS–NR array photoanodes with similar film thickness of 16 μm (inset is the simulated equivalent circuit). ( c ) Schematic demonstrations of electron transfer pathways for individual TNW, TNW–NS and TNW–NS–NR, respectively. Full size image The schematic illustrations of the electron transfer pathway (ETP) within TNW, TNW–NS and TNW–NS–NR can be seen in Fig. 5c . In particular, the TNW possesses the most direct ETP to facilitate electron transport. While for the TNW–NS–NR, a prolonged ETP is clearly evidenced mainly owing to the fact that the photoinjected electrons are not easily concentrated from dendritic NR as well as NS leaves to TNW stems within such a complicated network. In addition, a lower electron diffusion coefficient ( D n , D n = d 2 /(4 τ d )) [45] is obtained from the TNW–NS–NR cell ( Supplementary Fig. 5 ). As for the electron lifetime, short τ r for TNW–NS–NR indicates that the photo-generated electrons are more easy to attenuate before reaching the electrode, once they suffer a recombination with oxidized species of dyes or electrolytes [46] . However, as shown in Supplementary Fig. 6 , the electron diffusion lengths ( L n , L n =( D n τ r ) 1/2 ) [47] of the cells derived from all the TiO 2 arrays are >30 μm, which is much longer than the actual film thickness (16 μm) used in this study, demonstrating that the generated electrons can reach the electrode efficiently without overwhelming loss, and hence, we expect that much thicker films of such TiO 2 arrays can be fabricated to further enhance the photovoltaic performance without lowering their charge-collection efficiencies. To obtain better insight into the interfacial charge transfer resistances within DSSCs, electrochemical impedance spectroscopy characterization is carried out. Figure 5b shows the Nyquist plots of the DSSCs based on various TiO 2 architectures. According to a simulated equivalent circuit, charge transfer resistance ( R 2 ) at the TiO 2 /dye/electrolyte and corresponding electron lifetime ( τ r , τ r = R 2 × CPE2 (CPE2, chemical capacitance)) values are calculated [48] and then listed in Supplementary Table 5 . The R 2 values decrease significantly from 158.1 Ω for TNW to 65.08 Ω for TNW–NS, and then further decline to 30.98 Ω for TNW–NS–NR-based DSSCs, illustrating a faster recombination rate within DSSCs based on the latter two photoanodes with hierarchical structures. This is because the enlarged surface area of TNW–NS and TNW–NS–NR films provides more trapping sites for charge recombination with I 3 − in the redox electrolyte. The shortest electron lifetime (38.2 ms) for TNW–NS–NR hyperbranched array cells can be primarily attributed to the high germination density of the NSs anchoring sites and NR branches, which yields the maximum surface area, and in turn offers a high number of interfaces among TNW, TNS and TNR constituents, and thus generating numerous boundaries and defects for unexpected charge recombination [20] . The gradual decline of τ r for the three types of cells (from 87.5 to 38.2 ms) is in concurrence with the continuous reduction in V oc (from 870 to 812 mV) displayed in J-V results. Meanwhile, the dark current ( Supplementary Fig. 7 ) and open-circuit voltage decay ( Supplementary Fig. 8 ) measurements are also conducted to evaluate the charge recombination process. The larger dark current and faster voltage decay rate for TNW–NS–NR devices illustrate the parallel results of more serious charge recombination within these cells. In conclusion, a new approach of engineered integration and assembly of three well-defined constitutional units, that is, NWs, NSs and NRs into a complex 3D hierarchical monoblock has been successfully developed for the first time, via a full-solution-processed manner. Accordingly, hierarchically structured TiO 2 hyperbranched arrays composed of lamellar NSs on the NW stems with numerous elongated and cross-linked NR branches on all sides of the NSs and NWs were produced by sequential acid-thermal and hydrothermal processings on aligned smooth TiO 2 arrays. The DSSCs fabricated with TNW–NS–NR hyperbranched arrays yield a rather high energy conversion efficiency of 9.09%, which is the highest value observed for devices based on NW photoelectrode with similar film thickness and much higher than that of 1D smooth TNW scaffold (5.15%). The significantly improved efficiency was a direct consequence of maximized light-harvesting efficiency, originating from synergistic effects of greatly enhanced surface area for anchoring large amounts of dye molecule and superior light trapping and scattering for promoted light utilization efficiency. In a nutshell, the strength of current work lies in the scrupulous design of complex metal oxide array architectures and smart hybridization of specific nanounits (NWs, NSs and NRs) into a high-quality tree-like hyperbranched array with 3D interconnected networks by means of a simple and easy-to-operate full-solution-processed strategy, and the cells based on such a hyperbranched array photoanode do exhibit significantly enhanced efficiency. Most importantly, this work fully taps the greatest potential of NW-based electrodes, which is inspired by the motivation of taking full advantage of omnidirectional exploitation of geometry space of the oriented materials and thus maximizing omnidirectional light harvesting of array architectures in a broader wavelength range of incident light. However, there is still plenty of scope for further boosting the overall performance within such hyperbranched array systems. Some limitations of this study rest with the following issues. On one hand, the insufficient length of the arrays would limit the light-harvesting efficiency and thus restrict further improvement of overall power conversion efficiency. Hence, much effort should be paid on the optimized experimental details to increase the length of TNW arrays. On the other hand, it is well known that in addition to the performance of TiO 2 photoanode, other factors including panchromatic sensitizers with enhanced light harvesting, redox shuttles for reduced free energy loss as well as assistant catalysts for accelerating the sensitizer regeneration are all closely related to the overall device performance. Although such hyperbranched array architectures are solely applied in the conventional N719 sensitized solar cells with I − /I 3 − redox couple electrolyte and Pt catalyst in current study, we confidently believe that the effectiveness of our engineered TNW–NS–NR hyperbranched array architectures can be fully embodied if it is combined with a more efficient system composed of effective panchromatic sensitizer (that is, porphyrin dye, perovskite or narrow band gap quantum dots) or redox mediator (that is, solid-state or quasi solid-state electrolyte). Moreover, such vertically aligned anatase TNW–NS–NR hyperbranched arrays are anticipated to exhibit great significance and will emerge as a promising foundation in a wide range of applications such as sensing, photocatalysis, water splitting, optoelectronics, field emission, energy conversion and storage in the near future. Hyperbranched array architecture synthesis The TiO 2 -coated fluorine doped tin oxide (FTO) substrates were placed at an angle against the wall of the Teflon-lined stainless steel reactor containing a mixture of 0.4 g of PTO, 5 ml of deionized water (H 2 O) and 15 ml of DEG, and the reactor was then kept at 180 °C for 3 h for the growth of parental TNW array scaffold. The TNW samples were washed with ethanol, dried in air, followed by second-step acid-thermal reaction to construct epitaxial TNS on TNW. In a typical synthesis, 0.5 ml of TTIP was added into 30 ml of acetic acid (HAc) drop by drop and stirred for 30 min. The TNW sample on FTO glass was then introduced to the above solution and heated to 150 °C for different lengths of time (from 1 to 12 h). After the reaction, the TNW–NS sample was taken out and rinsed extensively with ethanol and water, followed by subsequent hydrothermal growth of TNR branches. In brief, the TNW–NS sample was loaded into the sealed reactor containing 0.35 g of PTO, 2.5 ml of H 2 O and 17.5 ml of DEG, and once again heated to 180 °C for different durations of time (from 1.5 to 9 h). The obtained films finally undergo an annealing treatment at 500 °C for 1 h to improve the crystallinity and remove the residual organics. Solar cell fabrication For use in DSSCs, different TiO 2 array samples were sensitized in a 0.5-mM N719 dye solution in acetonitrile/tert-butanol (1:1 v/v) for 16 h at ambient temperature. The TiO 2 working electrode was assembled into a sandwich-type cell together with Pt sheet counter electrode with the internal space of the device filled with a I − /I 3 − redox electrolyte by the capillary effect. Characterization The photovoltaic performances of the DSSCs were measured with active TiO 2 area of 0.16 cm 2 using a Keithley 2400 source meter under simulated AM 1.5G illumination (100 mW cm −2 ) provided by a solar light simulator (Oriel, model: 91192). The IPCE was measured on the basis of a Spectral Products DK240 monochromator as a function of wavelength from 400 to 800 nm. The electrochemical impedance spectra were obtained with a Zennium electrochemical workstation (ZAHNER) with the frequency range from 10 mHz to 1 MHz in the dark condition. IMPS and IMVS were also carried out on a electrochemical workstation (Zahner, Zennium) with a frequency response analyzer under a modulated green light emitting diodes (457 nm) driven by a source supply (Zahner, PP211), which can provide both DC and AC components of the illumination. The frequency range was set from 100 KHz to 0.1 Hz. Specifically, IMPS was measured under the short-circuit condition and the IMVS was measured under the open-circuit condition. The XRD patterns of the film samples on FTO glass slides were detected by XRD (Bruker D8 Advance). The morphological structure of the nanomaterials was directly characterized by field emission SEM (JSM-6330F) and TEM (JEOL-2010 HR). The total and diffuse transmittances as well as diffused reflectance spectra of TiO 2 arrays were measured on a UV/Vis-NIR spectrophotometer (UV-3150) with an integrating sphere to qualify the light scattering, reflecting and trapping of the samples. The amount of adsorbed dye was determined by immersing the films in 0.1 M of NaOH aqueous solution, and monitoring the concentration of desorbed dye by a UV/Vis-NIR spectrophotometer (UV-3150). How to cite this article: Wu, W.-Q. et al. Maximizing omnidirectional light harvesting in metal oxide hyperbranched array architectures. Nat. Commun. 5:3968 doi: 10.1038/ncomms4968 (2014).